Aerosol generation by raindrop impact on soil Aerosols are investigated because of their significant impact on the environment and human health. To date, windblown dust and sea salt from sea spray through bursting bubbles have been considered the chief mechanisms of environmental aerosol dispersion. Here we investigate aerosol generation from droplets hitting wettable porous surfaces including various classifications of soil. We demonstrate that droplets can release aerosols when they influence porous surfaces, and these aerosols can deliver elements of the porous medium to the environment. Experiments on various porous media including soil and engineering materials reveal that knowledge of the surface properties and impact conditions can be used to predict when frenzied aerosol generation will occur. This study highlights new phenomena associated with droplets on porous media that could have implications for the investigation of aerosol generation in the environment. Aerosols, which are tiny liquid droplets or solid particles suspended in a gas [1] , [2] , [3] , have been investigated because of their significant impact on the environment, human health and industrial applications [4] , [5] , [6] , [7] , [8] , [9] , [10] , [11] , [12] , [13] , [14] . Aerosol particles, larger than 1 μm, are known to originate from windblown dust and sea salt from sea spray resulting from bursting bubbles [6] , [15] , [16] , [17] , [18] , [19] , [20] . In addition, environmental aerosols are generated from both natural sources and anthropogenic activities such as volcanoes and combustion of fuels, respectively [3] . However, to the best of our knowledge, aerosol generation from raindrops hitting soil has not been reported and the origins of atmospheric bioaerosols containing elements of soil and environmental microorganisms remain illusive [1] , [8] , [21] . Aerosols generated from droplets hitting porous media can have significant impact on industrial applications as well as the environment [22] , [23] , [24] . There are several methods to generate aerosols such as electrospray, ultrasound and sprays; however, most methods use external energy sources to generate aerosol droplets. Because drop impingement-based aerosol generation can be employed using gravitational potential, it is promising for low-cost biological and environmental applications. Furthermore, this work could have widespread implications ranging from remediating the spread of disease-causing microbes to the earthy smell known as ‘petrichor’ present after a rain shower on a hot day [25] . In this work we provide evidence that rainfall on soil can also generate aerosols. High-speed imaging provides visual proof of aerosol generation when liquid water droplets hit soil at velocities consistent with rainfall. Within a specified range of impact velocities, we observe frenetic bubble generation and ejection of tiny droplets, producing aerosol above the surface ( Supplementary Movie 1 ). We can predict when the frenetic aerosol generation occurs from the surface properties and impact conditions. This work demonstrates that aerosols can be generated on porous surfaces including soil when impinged by a liquid droplet. Aerosol generation from droplets hitting soils Using different impact velocities, we observed drop impingement on soils using a high-speed camera ( Fig. 1a–c ; Supplementary Movie 2 ). When small water droplets, similar in size to raindrops, impinge on clay, sandy clay and clay loam [26] , aerosol generation is observed. As reported in ref. 20 , the diameter of a typical raindrop is 1–3 mm. The shape of a raindrop is not always spherical [27] , [28] , [29] because of the deformation in flight, but an assumed spherical shape is not unreasonable [30] . When a droplet hits the clay loam soil surface at a velocity consistent with light rainfall [31] ( Fig. 1a ), trapped gas bubbles appear inside the droplet ( Fig. 1b ). When the bubbles burst, multiple tiny jets of order tens of micrometres in diameter are ejected from the soil ( Fig. 1c ). It is believed that the bubbles pinned on the soil surface break when the bubbles reach the upper surface of the impinging droplet, resulting in bubble-bursting and liquid jets, a well-known occurrence during rainfall on the oceans, carbonated beverages and other problems in fluid dynamics [32] , [33] , [34] , [35] , [36] , [37] . 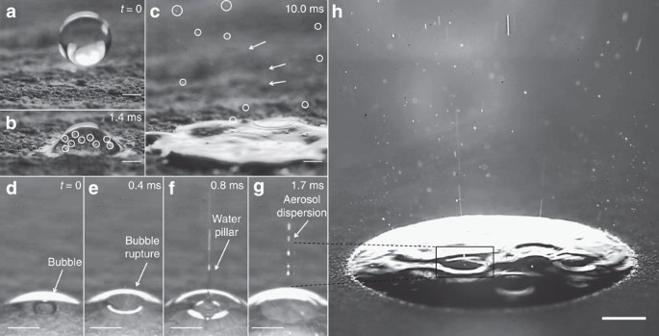Figure 1: Aerosol generation from droplets hitting soils and porous surfaces. (a) Clay loam with a rough surface before impingement with a droplet travelling at a speed of 2 ms−1. (b) Tiny bubbles form under the droplet after impact (delineated by white circles in the image). (c) Tiny water jets are ejected from the droplet after impact. Scale bars ina–c, 1 mm. The white circles and arrows in the image highlight aerosols and jets ejected from the droplet. (d–g) High-speed images of the aerosol-generation process when a single bubble breaks inside the droplet. Scale bars, 1 mm. (d) A bubble is trapped inside the droplet. (e) The bubble breaks at the droplet/air interface. (f) A water jet emanates from the droplet. (g) The jet breaks up into tiny droplets. (h) Frenetic water jets and associated aerosols are generated on a thin layer chromatography plate after impact with a droplet travelling at 1.4 ms−1. Scale bar, 1 mm. In the image, the white dots and lines are micron-scale water droplets ejected from the droplet on the surface. SeeSupplementary Movies 2–4. Figure 1: Aerosol generation from droplets hitting soils and porous surfaces. ( a ) Clay loam with a rough surface before impingement with a droplet travelling at a speed of 2 ms −1 . ( b ) Tiny bubbles form under the droplet after impact (delineated by white circles in the image). ( c ) Tiny water jets are ejected from the droplet after impact. Scale bars in a – c , 1 mm. The white circles and arrows in the image highlight aerosols and jets ejected from the droplet. ( d – g ) High-speed images of the aerosol-generation process when a single bubble breaks inside the droplet. Scale bars, 1 mm. ( d ) A bubble is trapped inside the droplet. ( e ) The bubble breaks at the droplet/air interface. ( f ) A water jet emanates from the droplet. ( g ) The jet breaks up into tiny droplets. ( h ) Frenetic water jets and associated aerosols are generated on a thin layer chromatography plate after impact with a droplet travelling at 1.4 ms −1 . Scale bar, 1 mm. In the image, the white dots and lines are micron-scale water droplets ejected from the droplet on the surface. See Supplementary Movies 2–4 . Full size image Observation of aerosol generation on porous media We first observed this phenomenon during drop impingement of liquid water on thin layer chromatography (TLC) plates. TLC plates can be considered ideal soil-like surfaces; they have similar water-absorption properties but they are topologically and chemically homogenous ( Table 1 ). For example, when a water droplet at a speed of 0.4 ms −1 hits a TLC plate with similar water-absorption properties as clay, a large bubble was trapped inside the droplet ( Fig. 1d ). When the bubble bursts ( Fig. 1e ), a thin water jet emerges ( Fig. 1f ). Then, the jet breaks up into small droplets, which remain suspended in air ( Fig. 1g ) ( Supplementary Movie 3 ). Frenetic water jets (aerosol dispersion) are observed in a specific range of impact velocities and surface properties, as shown in Fig. 1h ( Supplementary Movie 4 ). In this case, hundreds of water jets were ejected from the droplet at speeds of ~10 ms −1 in roughly 20 μs. Table 1 Characteristics and wetting properties of the media used to examine aerosol generation. Full size table Delivery of materials in porous media with aerosols From the environmental perspective, an aerosol refers to tiny suspensions that possess chemicals or solid particles [3] . Therefore, it is important to verify that materials within the porous media are entrained into the aerosols generated from droplets hitting porous media. To confirm that materials are transported with the aerosol, we conducted drop impingement on porous media with Rhodamine B on the pores. If the dye is suspended in the aerosol droplets, this can be observed under ultraviolet illumination. In a duct with a low-speed air flow, aerosols were generated from water (deionized water) droplets hitting porous surfaces permeated with Rhodamine B. Transparent glass is located above the porous media to collect the aerosol droplets generated from the porous media ( Supplementary Fig. 1 ). The number of fluorescent spots on the transparent glass was measured with respect to distance from the location of aerosol generation. With increasing air-flow velocity, the mean of the particle distribution shifted away from the position of aerosol generation ( Supplementary Fig. 2 ). This result shows that particulate matter within the porous surface can be convectively dispersed as aerosols generated from drop impingement. Aerosol-generation process Aerosol generation after drop impingement on porous media is a three-step process consisting of bubble formation, bubble growth and bubble bursting, as shown in Fig. 2 . We performed experiments with different impact velocities and surfaces in order to elucidate the aerosol-generation mechanism ( Supplementary Movies 5–7 ). High-speed images shown in Fig. 2a–c reveal the aerosol-generation process shown schematically in Fig. 2d–g . When a droplet hits the surface, the droplet flattens because of its kinetic energy. Tiny bubbles are trapped at the droplet/surface interface because the droplet expansion speed is faster than the water-absorption speed of the surface ( Fig. 2d ). It is known that a thin air film, with thickness 1 μm, forms on a flat surface when surface roughness is less than 2 nm (root-mean-square, RMS), for Weber number (We) from 700 to 900 and Re from 1,600 to 5,800 (refs 38 , 39 ). Subsequently, the air film evolves into a single bubble. On rough surfaces, the air film can be fragmented into small bubbles because of the irregularity of the surface. The period of the air film retraction is fast, given it’s speed of roughly 5 ms −1 (ref. 39 ). The time required to form small air bubbles inside the droplet is shorter than hundreds of microseconds [39] . Compared with the bubble formation, the speed of droplet absorption into porous media is much slower because the porous media and soils, used in this work, have hydraulic diffusivities lower than 1.5 × 10 −4 m 2 s −1 ( Table 1 ). A thin air film forms on rough surfaces such as soils during impact, and then fragments into small bubbles because of the irregularity of the porous surfaces during the air film retraction. The bubbles grow with air supplied from the porous media as it absorbs the liquid and displaces trapped air ( Supplementary Movies 5 and 6 ). After the droplet reaches its maximum radius, the droplet oscillates, relieving its compressive pressure. At this time, bubbles grow by receiving air escaping from the pores of the surface as water is absorbed ( Fig. 2e ). The droplet height above the surface is reduced as the liquid enters the porous media ( Fig. 2f ). Finally, the bubbles burst when they meet the air–water interface of the droplet ( Fig. 2g ), ejecting small jets that breakup into tiny droplets. 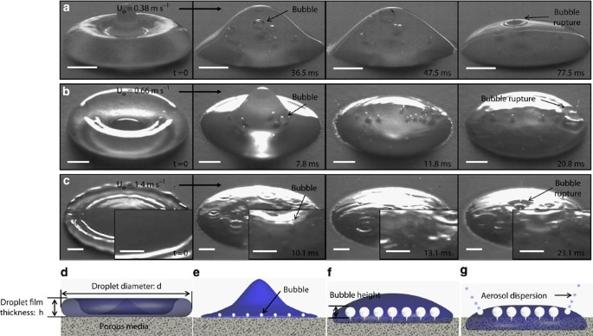Figure 2: Three-step process of aerosol generation after drop impingement on porous media. (a–c) High-speed images of bubble formation inside water droplets on a thin layer chromatography plate, composed of aluminium oxide particles (11–14 μm), with respect to impact velocity (Uo). Scale bars, 1 mm. (d–g) Schematic illustration of the aerosol-generation process. (d) A droplet influences a porous surface and expands. (e) After the droplet reaches maximum diameter, tiny bubbles are entrained at the interface of the droplet and the porous surface. (f) The droplet height decreases as water absorbs into the porous surface, while the bubbles grow due to air trapped in the porous surface. (g) Bubbles meet the air/water interface and rupture, generating tiny water jets. The number of bubbles created inside the droplet increases with impact velocity. SeeSupplementary Movies 5–7. Figure 2: Three-step process of aerosol generation after drop impingement on porous media. ( a – c ) High-speed images of bubble formation inside water droplets on a thin layer chromatography plate, composed of aluminium oxide particles (11–14 μm), with respect to impact velocity ( U o ). Scale bars, 1 mm. ( d – g ) Schematic illustration of the aerosol-generation process. ( d ) A droplet influences a porous surface and expands. ( e ) After the droplet reaches maximum diameter, tiny bubbles are entrained at the interface of the droplet and the porous surface. ( f ) The droplet height decreases as water absorbs into the porous surface, while the bubbles grow due to air trapped in the porous surface. ( g ) Bubbles meet the air/water interface and rupture, generating tiny water jets. The number of bubbles created inside the droplet increases with impact velocity. See Supplementary Movies 5–7 . Full size image To generate aerosols from drop impingement on porous media, bubbles must form inside the initial large droplet after impact. In this work we consider droplets hitting dry soil, which is both wettable and firm enough to maintain its porous structure during the impingement. When droplets have an impact on powder surfaces or granular layers [40] , [41] , [42] , [43] , [44] , we did not observe bubble formation during the drop impingement. We speculate that if the porous media deform considerably during impact there are low permeability paths for air to escape from beneath the droplet and so it is not trapped. However, more investigation is needed to justify this claim and illuminate the relationship between aerosol generation and mechanical strength of porous media. Effects of impact conditions on aerosol generation From the relationship between the kinetic energy and the surface energy of the droplet, we can estimate the size and number of bubbles after impact. It is known that jet diameter and velocity are strongly correlated with bubble size [15] , [34] , [45] . Previously, we have shown using energy conservation that the maximum diameter of a droplet after impact is linearly proportional to the impact velocity [46] . Therefore, the minimum droplet height (the droplet film thickness when the droplet reaches its maximum diameter after impact, Fig. 2d ) is inversely proportional to the square of impact velocity as follows: U o 2 ~ d max 2 ~ h min −1 , where U o is the impact velocity, d max is the maximum droplet diameter and h min is the minimum droplet film thickness ( Fig. 3a ). Therefore, impact velocity governs the maximum bubble size inside the droplet because bubble size cannot exceed the droplet film thickness. 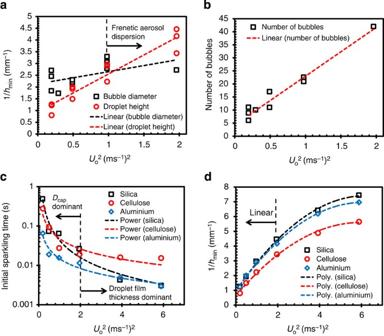Figure 3: Characteristics of droplets and bubbles generated after impingement on TLC plates. The hydraulic diffusivities of TLC-A (silica), TLC-B (cellulose) and TLC-C (aluminium) are 9.5, 20.4 and 22.4 mm2s−1, respectively. The dot lines indicate the fitting lines of the experimental data marked with symbols. (a) The average bubble diameter does not change significantly with impact velocityUo2but the average droplet film thickness is inversely proportional toUo2. (b) The maximum number of bubbles inside the droplet linearly increases with respect toUo2. (c) The time it takes to observe the first jet is affected by the surface wettability at low impact velocity but by the droplet film thickness at high impact velocity, since the droplet film thickness governs the maximum bubble size at high impact velocity. (d) The droplet film thicknesshminafter hitting the surfaces is the highest on TLC-B. Figure 3: Characteristics of droplets and bubbles generated after impingement on TLC plates. The hydraulic diffusivities of TLC-A (silica), TLC-B (cellulose) and TLC-C (aluminium) are 9.5, 20.4 and 22.4 mm 2 s −1 , respectively. The dot lines indicate the fitting lines of the experimental data marked with symbols. ( a ) The average bubble diameter does not change significantly with impact velocity U o 2 but the average droplet film thickness is inversely proportional to U o 2 . ( b ) The maximum number of bubbles inside the droplet linearly increases with respect to U o 2 . ( c ) The time it takes to observe the first jet is affected by the surface wettability at low impact velocity but by the droplet film thickness at high impact velocity, since the droplet film thickness governs the maximum bubble size at high impact velocity. ( d ) The droplet film thickness h min after hitting the surfaces is the highest on TLC-B. Full size image The number of bubbles and their diameter can be measured from the high-speed images ( Fig. 3a,b ). We find that the number of bubbles is proportional to the wetted area of the surface, which can be calculated from the maximum diameter of the spreading droplet. The relationship between the maximum number of bubbles and the impact velocity is as follows: U o 2 ~ A max ~ N max, where A max is the maximum wetted area of the surface, and N max is the maximum number of bubbles formed inside the droplet ( Fig. 3b ). We employ the Weber number, We= ρd o U o 2 γ −1 , to evaluate the effect of impact velocity on the number of bubbles and the bubble size, where ρ is the liquid density, d o is the initial droplet diameter and γ is the liquid surface tension. Effects of wetting properties on aerosol generation The droplet permeation and the initial aerosol dispersion are affected by surface properties, mainly the wettability. The water-absorption speed of porous media can be characterized by the hydraulic diffusivity, D cap = r c γ cos θμ −1 , and r c is the effective capillary radius, θ is the native contact angle of surface and μ is dynamic viscosity of the liquid [47] . If we assume that dry soil becomes fully wet after capillary suction (for example, there are no impenetrable pores), the hydraulic diffusivity can be found using the equation for capillary rise in the absence of gravitational effects: H 2 ~ D cap t , where H is the rise height and t is time [48] , [49] , [50] . The hydraulic diffusivity can be experimentally estimated from capillary rise measurements [50] . We now define a modified Péclet number (Pe=( U o d o ) D cap −1 ). The modified Péclet number is the ratio of the advective transport rate ( U o d o ) to the hydraulic diffusivity ( D cap ) and used to represent the effects of surface wettability. Figure 3c,d shows the effects of surface wettability and impact velocity on aerosol generation. In Fig. 3c , jetting initiation time is the time it takes to observe the first aerosol dispersion after the droplet reaches the maximum diameter after impact. The jetting initiation time is mainly governed by the wetting properties of the surface at low impact velocity ( Fig. 3c ). However, the droplet film thickness significantly affects the jetting initiation time at high impact velocities. TLC-A and TLC-C have the lowest and the highest hydraulic diffusivities, respectively. Therefore, the initial jetting occurs on TLC-C first and on TLC-A last at low impact velocities (less than 1.4 ms −1 ). At higher impact velocities (higher than 2.0 ms −1 ), however, the droplet height is the highest on TLC-B, as shown in Fig. 3d ; therefore, the jetting initiation time is highest on TLC-B. Effect of porous structures on aerosol generation Repeated drop impingements, which can fill up the pores with water, were conducted to examine the effect of porous structures. First, we periodically released water droplets within a period of 10 s. In this case, aerosol generation was not observed after the second drop impingement. However, when the period was 5 min, aerosol generation was observed in every drop impingement. These experiments show that bubbles are formed at the droplet/surface interface due to the inflation with air stored in pores of the surfaces. If the pores are filled with liquids, bubbles cannot form, resulting in no aerosol generation after impact. However, after the pores are dry, bubbles can be trapped again at the droplet/surface interface and generate aerosol when the bubbles break. It has been reported that bubbles can be generated and entrained in a droplet within the drop impact on solid and liquid [51] , [52] . However, the result of repeated drop impingements reveals that thin air films trapped at the droplet/solid or droplet/liquid interface is not the main reason of aerosol generation from droplets hitting porous surfaces. Inflation of air from porous structures has the important role of aerosol generation. From Table 1 , surface roughness of the porous media and soils used in this work ranges from 1 to 60 μm. Interestingly, aerosol generation was observed for surface roughness (RMS) ranging from 1 to 10 μm. This range is slightly higher than the air film thickness (1 μm) formed on solid surfaces during impact [38] , [53] . From this information we can speculate as to why aerosol is not generated on highly roughened surfaces. First, thin air films cannot form on surfaces with high surface roughness exceeding roughly 10 μm; therefore, small bubbles are not trapped on the surfaces during the air film retraction. Second, higher surface roughness has a tendency to increase the effective pore radius of the porous media, resulting in higher hydraulic diffusivity [50] . Indeed, air bubbles were not observed on porous media with hydraulic diffusivity and surface roughness higher than 50 mm 2 s −1 and 20 μm, respectively. Characterization of aerosol generation On the basis of the drop impingement results, we found a domain that resulted in aerosol generation. We employ the We and a modified Péclet number (Pe) parameters in a two-dimensional (2D) map of our experimental conditions. We observed drop impingements on various types of porous media, including soils, with different liquids and impact velocities. In total we conducted roughly 600 experiments. Experiments were performed on 16 different soils (eight commercial soils purchased from World’s Science, and other soils collected from the Boston metropolitan area), five different TLC plates (Sigma-Aldrich, micro- and nanoporous surfaces: silica, cellulose and aluminium oxide with different pore sizes) and seven porous titania films fabricated in-house [50] (microporous surfaces fabricated with different conditions) with four different liquids (water, ethanol, ethylene glycol and glycerol; Table 1 ). 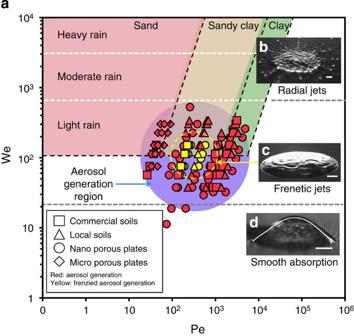Figure 4: Characterization of aerosol generation when droplets hit soils and porous surfaces. (a) Thexaxis indicates a modified Péclet number (Pe≡(Uodo)/Dcap), whereUoanddoare the impact velocity and the diameter of the droplet. Theyaxis indicates the Weber number (We≡ρdoUo2γ−1), mainly varied by the impact velocity. We and Pe represent the impact condition and the surface property, respectively. TheDcapvalues of the soils were measured by the capillary rise experiments. The red symbols indicate the observation of aerosol dispersion from the droplets at the corresponding We and Pe. The blue circle indicating ‘aerosol-generation region’ highlights the group of the data points (the red symbols) where aerosols are generated. The yellow symbols inside the aerosol-generation region show the data points resulting in frenetic aerosol generation. Rainfalls on soils are placed on the upper part of the characterization map, and clay and sandy–clay soils have concentrated regions in the aerosol generation region. (b–d) The representative images of drop impingements in the regions classified with We. Scale bars, 1 mm. The horizontal dot lines and the diagonal dot lines indicate the constant We numbers and the constantDcapnumbers, respectively. Figure 4 summarizes the observations with respect to Pe and We. We and Pe were varied from 1 to 10 4 and from 1 to 10 6 , respectively. Aerosol generation is observed in a specific region of We and Pe, as shown in Fig. 4 . There was no aerosol generation in the low and high We regions (We<10 or We>10 3 ). When We>10 3 , we do not observe aerosol generation because splashing in radial direction ( Fig. 4a ) leads to air entrainment. By contrast, when We<10, few bubbles are entrained and they are much smaller than the droplet height, resulting in delayed bubble bursting and reabsorbed bubbles into the surface. In addition, the surfaces did not show aerosol generation at high or low hydraulic diffusivity (Pe<10 or Pe>10 4 ). When Pe>10 4 , bubbles cannot become sufficiently large to generate aerosols during droplet spreading because the droplet does not permeate into the surface. Conversely, if Pe<10, the droplet quickly absorbs into the porous surface, faster than the droplet expands. Therefore, air is not trapped at the interface of the droplet and the surface, and there is no aerosol generation. Figure 4: Characterization of aerosol generation when droplets hit soils and porous surfaces. ( a ) The x axis indicates a modified Péclet number (Pe≡( U o d o )/ D cap ), where U o and d o are the impact velocity and the diameter of the droplet. The y axis indicates the Weber number (We≡ ρd o U o 2 γ −1 ), mainly varied by the impact velocity. We and Pe represent the impact condition and the surface property, respectively. The D cap values of the soils were measured by the capillary rise experiments. The red symbols indicate the observation of aerosol dispersion from the droplets at the corresponding We and Pe. The blue circle indicating ‘aerosol-generation region’ highlights the group of the data points (the red symbols) where aerosols are generated. The yellow symbols inside the aerosol-generation region show the data points resulting in frenetic aerosol generation. Rainfalls on soils are placed on the upper part of the characterization map, and clay and sandy–clay soils have concentrated regions in the aerosol generation region. ( b – d ) The representative images of drop impingements in the regions classified with We. Scale bars, 1 mm. The horizontal dot lines and the diagonal dot lines indicate the constant We numbers and the constant D cap numbers, respectively. Full size image Frenetic aerosol generation is observed at the core of the aerosol-generation region on the characterization map (c.f. yellow symbols in Fig. 4 ). To achieve frenetic aerosol generation, bubbles must not only reach sufficient size to disperse aerosol but also become similar in size to the droplet film thickness in order to break simultaneously when the bubbles meet the top surface of the droplet. Therefore, moderate Pe (10 2 <Pe<10 3 ) is necessary for frenzied aerosol generation since this balances bubble size (favouring high Pe) while minimizing the time it takes for the initial droplet to spread and the bubbles to burst (favouring low Pe). According to the study by Lee et al. [34] , bubbles must have a minimum size to generate liquid jets when they burst. The average bubble height and the average droplet height become similar within a specific range of We ( Fig. 3a ). Frenetic aerosol generation occurs when the bubble diameter is very close to the droplet height, leading multiple bubbles to burst at roughly the same time after impact ( Fig. 4b ). As shown in Fig. 4 , frenetic aerosol generation occurs when We/Pe~1. In previous work, we defined We/Pe=Re W = U o ρr c cos θμ −1 , where Re W is the Washburn–Reynolds number. Re W is the ratio of the droplet inertial to the capillary flow properties of the porous media as We/Pe= ρD cap U o γ −1 like the capillary number with ρD cap replacing μ . This frenetic aerosol dispersion is very attractive because quite a number of aerosols can be produced within a few microseconds, which could be useful for applications requiring fast aerosol generation at ambient temperature. It is well known that air films are trapped between droplets and solid surfaces during impact [38] , [39] , [51] , [54] , [55] . In general, the main features of drop impact dynamics are described by We and Re. It has been reported that the splashing condition on a solid surface can be defined as K d =We 1/2 Re 1/4 >57.7 (refs 55 , 56 ). In this work, drop impingement was conducted for Re from 60 to 10,244 and K d from 7 to 325. The frenetic aerosol-generation region, occurring at Re W ~1, corresponds to K d ~70 and Re~5,000. In our previous work [46] , the splashing region (radial jetting) can be characterized as Re W >5, which corresponds to K d >100. Frenetic aerosol generation occurs at slightly lower Re W than what is required for splashing. This result shows reasonable agreement with the other drop impingement studies because the splashing starts around K d ~70. The advantage of using Re W is that we can consider the impact conditions and the wetting properties simultaneously. Therefore, we can predict impingement modes considering various kinds of surfaces with a wide range of wetting properties. Re W can be used to predict the patterns of aerosol dispersion from droplets. Interestingly, when Re W =We/Pe<0.2, we observe aerosol dispersion at the edge of droplets. Supplementary Movie 8 shows edge aerosol dispersion when a silica TLC plate was used as the substrate with We=113 and Pe=501. This aerosol dispersion has a different mechanism from that of jets originating from the cusps of droplets hitting flat surfaces at relatively high impact velocity [55] , [57] . For the case of drop impingement on flat surfaces, Yarin et al. [57] suggested the dimensionless impact velocity u =Ca λ 3/4 = U o ( ργ −1 ) 1/4 v −1/8 f −3/8 , where Ca is the capillary number, v is the kinematic viscosity and f is the drop frequency, to predict the splashing threshold. The splashing threshold is defined when u =17–18 under the assumption that surface roughness is much less than droplet diameter. We cannot estimate the dimensionless impact velocity in our cases because we used a single droplet for the drop impingement rather than using successive droplets with drop frequency f . Compared with the minimum impact velocity of 5 ms −1 for splashing in successive drop impingement, we observe the side aerosol dispersion for impact velocities lower than 2 ms −1 . Edge aerosol dispersion occurs when the maximum bubble size is smaller than the droplet height. Under this condition the bubbles begin bursting at the edge of the droplet. We observe aerosol dispersion at the edge of droplets on both smooth and rough porous surfaces, as shown in Supplementary Movies 2 and 8 , respectively. From the characterization map we conclude that aerosol generation can occur during light and moderate rainfall on soils with hydraulic diffusivity less than sand. To locate the impingement domains for rainfall on soil (red, yellow and green regions in Fig. 4 ), the hydraulic diffusivity of the soils were obtained from the literature [58] , [59] , [60] and the impact velocity of raindrops was set from light rain ( U o <4.0 ms −1 ) to heavy rain ( U o >7.0 ms −1 ) [31] . When the impingement domains are added to the characterization map, the overlapping regions of aerosol generation and rainfall are evident ( Fig. 4 ). We verified aerosol generation experimentally for conditions consistent with light and moderate rain on soil with similar water-absorption properties as clay and sandy clay soil. Aerosol generation was not observed on sand or during conditions consistent with heavy rainfall. In this work we demonstrate that aerosols can be generated from raindrops on soil. However, there are a few limitations of this work that have yet to be fully explored. First, raindrop–aerosol collisions are a major mechanism of aerosol removal [3] . Even though aerosols are generated from droplets, successive raindrops can eliminate the aerosols from the air; therefore, large-scale environmental effects might not be expected. Second, the gravitational settling velocity can be relatively fast when the droplet size is around a few tens of microns. Even when considering evaporation, the settling speed is not negligible. Therefore, further investigation of aerosol migration is necessary to understand the potential for large-scale environmental effects of aerosols generated on soil. One mechanism that could enhance the relevance of this phenomenon is wind-driven advection. Considering wind on the surface of porous media, tiny droplets or solid particles (<50 μm) can be transferred very long distances from the origin, up to a few thousand kilometres [61] , [62] . Furthermore, aerosols can have higher velocities than raindrops because of their small size, leading to lower inertia and drag forces [24] , [30] . Therefore, aerosols have the potential to migrate long distances without serious washing out or gravitational settling. In this manuscript, we focused on a novel mechanism of aerosol generation from droplets hitting porous media rather than exploring the effects of the aerosols. This discovery will lead to additional work investigating the fate of these aerosols in the environment. This work has at least two unique contributions: first, we present visual evidence of aerosol generation from rainfall on soil; and second, we provide an effective means to generate aerosol using simple drop impingement on porous media. The results of this work indicate a strong correlation between aerosol generation, wetting properties and droplet impact velocity. Now that this phenomenon has been observed, future work could explore the environmental effects of aerosol generation on soil. In addition, results of this study could be used to develop novel chemical synthesis methods for next-generation materials employing aerosols [63] . This work could also be utilized to study the transport of viruses and bacteria impregnated in soil. Measurements of hydraulic diffusivity In this study, capillary rise measurements [64] , [65] , [66] were performed to evaluate hydraulic diffusivity on porous surfaces and soils ( Table 1 ). For the capillary rise measurements of soils, we used a common experimental set-up used in previous work [60] , [64] , [66] . A glass tube, with 10 mm inner diameter, is filled 100 mm of soil and capped at the bottom with a glass membrane. The pore size of the membrane is in the 70- to 100-μm range. The glass tube is fixed vertically and the liquid bath height is slowly increased to initiate contact between the soil sample and the liquid surface. Capillary rise is recorded using a digital camera. For capillary rise measurements on the other surfaces, the samples, which measured 2 cm in width and 10 cm in length, were used instead of glass tubes. Theoretical determination of hydraulic diffusivity Hydraulic diffusivity was originally derived from Darcy’s law; therefore, we need to understand how the hydraulic diffusivity correlates with the capillary rise measurement. The hydraulic diffusivity obtained from the capillary rise measurement has the same physical meaning as the hydraulic diffusivity obtained from Darcy’s law, assuming a uniform porous structure. The following two sections describe the derivations of hydraulic diffusivity using both approaches. Hydraulic diffusivity from capillary rise measurements Capillary flows can be considered a subset of Poiseuille flow in a narrow tube with radius, r c . The velocity within a capillary can be written as where ∂P / ∂z is the pressure gradient in the z direction and μ is the liquid viscosity. In the tube, the capillary pressure, P cap , can be calculated from the Young–Laplace equation, where γ is the surface tension and θ is the native contact angle on the surface. If the capillary pressure is higher than the hydrostatic pressure in the capillary tube, the liquid rises. When a vertical capillary tube comes into contact with the free water surface, the flow velocity can be expressed by modifying equation (1). For a vertical tube with rise height, H , from the free liquid surface to the propagating liquid front, and the average velocity, v c , can be expressed as the change in capillary height with respect to time. Washburn’s equation, which is also attributed to Lucas [67] , and Bell and Cameron [68] , is obtained as [49] If H is small, gravitational effects can be neglected and Washburn’s equation can be simplified to Equation (4) can be integrated with respect to H and t to obtain a function relating rise height with time, resulting in the expression: where D cap is the hydraulic diffusivity with the units of m 2 s −1 . Therefore, hydraulic diffusivity can be obtained from experimental measurements of the capillary rise speed. Hydraulic diffusivity from Darcy’s law From Darcy’s law, the water discharge, q (ms −1 ), through porous media can be expressed as where K is the hydraulic conductivity (ms −1 ) and ∂P / ∂z is the hydraulic gradient in the z (or vertical) direction. When we assume the capillary head, H cap , is the only driving force for the water discharge, from equations (1) and (6), we can express the hydraulic conductivity as Assuming water content continuity, the Richards’ equation [47] , [69] can be derived from equation (6) as where Θ is the moisture content. Here capillary pressure is considered the only driving force; therefore, we can express equation (8) as a function of hydraulic diffusivity, D , as follows: where If we assume that the porous medium is initially dry (Θ=0) and becomes fully wet (Θ=1) after capillary suction, and the capillary pressure becomes zero when Θ=1, the hydraulic diffusivity when the porous medium is dry can be expressed as from equations (7) and (10). Therefore, the hydraulic diffusivities obtained from Washburn’s and Richard’s equations have the same form. Preparation and characterization of porous media We used 28 different porous medium samples (see Table 1 ) to examine aerosol generation from drop impingement. Eight kinds of soil (from clay loam soil to peat) were purchased from World’s Science (Nasco soil samples, Fort Atkinson, WI). We used the soil classification based on the product information provided by the company. Eight soil samples were collected from the Boston metropolitan area. The detailed soil sample locations are as follows; Soil A: Killian court on MIT campus, Soil B: Amherst Alley on MIT campus, Soil C and Soil D: Briggs field on MIT campus, Soil E, Soil F and Soil G: Charles River and Soil H: Nahant beach. The soils were classified considering the particle size and sampling location. In addition, we tested five kinds of commercial TLC plates purchased from Sigma-Aldrich, and seven different titania porous films produced by an electrochemical process [50] . To prepare soil substrates, first we gently broke the soils into fine grains by hand. We did not filter and grind the soils. Then, 1 cm of each soil was placed on a dish and then wetted with a water spray. The wetted soils were dried on a hot plate at 50 °C for 3 days. After cooling to room temperature, the soils were used for the drop impingement experiments. The TLC plates were used as provided from the manufacturer. The porous titania plates were rinsed with deionized water for 1 min after processing and dried at ambient conditions. From capillary rise experiments, the hydraulic diffusivity of each porous medium was evaluated with four different liquids: water, ethanol, ethylene glycol and glycerol. For the soils, the hydraulic diffusivity and aerosol generation were evaluated with water. The TLC and porous titania plates were evaluated with four different liquids: water, ethanol, ethylene glycol and glycerol. The particle sizes of the soil samples were evaluated using an image-processing and analysis software (ImageJ, US National Institutes of Health, Bethesda, MD, USA). Table 1 summarizes the surface properties and liquids used in this work. Characterization of drop impingement on TLC plates We investigated the behaviours of droplets hitting porous surfaces using high-speed imaging. We used the three different TLC plates (TLC-A, TLC-B and TLC-C), with wetting properties shown in Table 1 , and varied the drop height to change the impact velocity. First, we compared the droplet film thickness after spreading and the bubble diameters, as shown in Fig. 3a . The droplet film thickness is measured when the droplets reach their maximum radius after impact. The bubble diameter is the average diameter of the bubbles inside the droplet when the first bubble breaks. Delivery of materials in porous media with aerosol In a duct with air flow, aerosol was generated from deionized water droplets hitting porous surfaces containing a fluorescent dye (Rhodamine B, Sigma-Aldrich). First, we dropped Rhodamine B suspensions (2.1 × 10 −5 M) on TLC-C plates, which were then dried in a common laboratory environment for 1 day. The TLC plate was placed in a duct, with dimensions of 10 cm × 10 cm × 160 cm in width, height and length, respectively ( Supplementary Fig. 1a ). A transparent glass slide ( Supplementary Fig. 1b ) was placed at height h from the TLC plate to acquire aerosol droplets generated from the TLC plate. The transparent glass slide has a hole with the diameter of 5 mm to allow water droplets to hit the TLC plate. Using an electric fan, air flow was generated in the duct. After conducting drop impingement on the TLC surfaces ( Supplementary Movie 9 ), we observed the transparent glass slides with a microscope to count the number of the sites where aerosol droplets were deposited. If the aerosol droplets contain traces of chemicals initially on the porous surface, we would expect to observe Rhodamine B on the glass where the aerosol droplets hit. We used a microscope (Nikon Eclipse Ti) with a UV filter, with a centre excitation wavelength of 535 nm, to distinguish the sites with Rhodamine B. Under the microscope, the regions with Rhodamine B are relatively bright and easy to distinguish ( Supplementary Fig. 1c ). First, we measured the number of Rhodamine B spots on the glass slides, at three different heights: 2, 3 and 5 mm from the TLC plate, when aerosol was generated in the duct without air flow. Second, we used three different air-flow speeds: 0.125, 0.25 and 0.5 ms −1 to verify that chemicals on the porous media convectively migrate as aerosol droplets. We counted the number of Rhodamine B spots on the downstream half of the circle. How to cite this article: Joung, Y. S. & Buie, C. R. Aerosol generation by raindrop impact on soil. Nat. Commun. 6:6083 doi: 10.1038/ncomms7083 (2015).